Synthesis of tertiary alkylphosphonate oligonucleotides through light-driven radical-polar crossover reactions Chemical modification of nucleotides can improve the metabolic stability and target specificity of oligonucleotide therapeutics, and alkylphosphonates have been employed as charge-neutral replacements for naturally-occurring phosphodiester backbones in these compounds. However, at present, the alkyl moieties that can be attached to phosphorus atoms in these compounds are limited to methyl groups or primary/secondary alkyls, and such alkylphosphonate moieties can degrade during oligonucleotide synthesis. The present work demonstrates the tertiary alkylation of the phosphorus atoms of phosphites bearing two 2’-deoxynuclosides. This process utilizes a carbocation generated via a light-driven radical-polar crossover mechanism. This protocol provides tertiary alkylphosphonate structures that are difficult to synthesize using existing methods. The conversion of these species to oligonucleotides having charge-neutral alkylphosphonate linkages through a phosphoramidite-based approach was also confirmed in this study. Recently, oligonucleotides have attracted attention with regard to pharmaceutical applications. These compounds exhibit high specificity for certain molecules and can allow the delivery of small-molecule drugs and antibodies to targets that are otherwise challenging to access [1] , [2] . Although naturally-occurring oligonucleotides are susceptible to degradation by endogenous nucleases, the chemical modification of oligonucleotides can be used to mitigate this instability and provide pharmaceuticals with high specificity for mRNA and miRNA [3] , [4] . In fact, chemically-modified oligonucleotides have been approved and marketed over the last two decades [5] . Oligonucleotides are composed of contiguous nucleotide subunits each having a sugar-based scaffold, and so the phosphodiester backbones and nucleobases of these compounds have been examined as potential sites of chemical modification [6] , [7] . However, while a variety of sugar-modified nucleic acids have been developed, the range of backbone modifications remains limited. Chemical modifications of the phosphodiester backbone directly affect the metabolic stability of these compounds and also alter their pharmacokinetic profiles [8] . The formation of phosphorothioate (PS) groups is an example of a typical phosphodiester backbone modification and is found in the majority of commercially available oligonucleotide therapeutics [9] . This modification involves the replacement of the non-bridging oxygen atom in a phosphodiester bond with a sulfur atom as a means of increasing metabolic stability and lipophilicity. However, PS-modified oligonucleotides can exhibit toxicity as a consequence of nonspecific interactions between the negatively charged sulfur atoms and the positively charged proteins that are ubiquitous in living systems [10] . Charge-neutral backbone modifications are expected to maintain a high degree of metabolic stability while avoiding this toxicity. Present approaches to obtaining charge-neutral backbones comprise triester-type P–O linkages, several P–N linkages (such as phosphorodiamidate backbones in phosphorodiamidate morpholino oligomers (PMO) and phosphoranylguanidine backbones) and P–C linkages, such as in the case of methylphosphonate (MP) and methoxypropylphosphonate (MOP) moieties (Fig. 1A ) [5] , [6] , [11] . It should be noted that P–C backbones can be associated with challenges related to chemical stability, although high levels of nuclease resistance following the bonding of alkyl groups not found in natural products to phosphorus atoms has been demonstrated [12] , [13] . On this basis, we anticipated that sterically-hindered tertiary alkylphosphonates could serve as robust charge-neutral backbones ensuring high chemical stability. The conventional synthesis of oligomers containing P–C backbones involves the preparation of phosphoramidites in which a P–C bond is already introduced. However, to the best of our knowledge, there are presently no techniques for introducing bulky, multi-substituted carbon groups onto a phosphorus atom and then bonding this atom to a phosphoramidite. Moreover, steric hindrance effects might be expected to prohibit the use of tertiary alkylphosphonates in this coupling step. Because alternative approaches to oligonucleotide synthesis have not yet been unexplored, there is a need to develop a fundamentally different approach that is compatible with a high degree of steric hindrance and with a wide range of functional groups. Fig. 1: Chemical modification of oligonucleotides. A Applications of P–C backbones in oligonucleotide pharmaceuticals. MP methylphosphonate. MOP Methoxypropylphosphonate. B Carbocation generation via a light-driven radical-polar crossover mechanism. SET, single electron transfer. C Synthesis of oligonucleotides bearing tertiary alkylphosphonate backbones (this work). Full size image Carbocations are highly reactive and hence can be employed to attach bulky alkyl substituents to heteroatom centers [14] . However, present-day methods require the use of strong acids to generate the carbocation species, which limits the range of functional groups that can be accepted [15] . Newer electrochemical and photochemical approaches have enabled the generation of carbocations under milder conditions without the use of strong acids as a means of forging C(sp 3 )–heteroatom bonds with various heteroatom nucleophiles [16] , [17] , [18] , [19] , [20] . Our own group previously developed a light-driven radical-polar crossover (RPC) protocol that combines visible light-mediated photoredox catalysis with an RPC mechanism and requires only mild conditions (Fig. 1B ) [21] , [22] , [23] , [24] , [25] , [26] , [27] . In this process, a photo-excited benzo[ b ]phenothiazine donates an electron to a redox-active ester derived from a carboxylic acid in response to visible light irradiation to form a benzo[ b ]phenothiazine radical cation along with an alkyl radical, with the liberation of carbon dioxide. Subsequently, the alkyl radical is oxidized by the radical cation with the simultaneous combination of these species to form an alkylsulfonium compound. This alkylsulfonium species can subsequently react with a nucleophile, serving as a carbocation analogue. This method permits various tertiary and secondary alkyl substituents to be attached to heteroatom nucleophiles without the use of strong acids, such that a number of different highly functionalized molecules can be obtained. We envisioned that the carbocation equivalent (that is, the alkylsulfonium) generated by the light-driven RPC protocol could be applied to the tertiary alkylation of the phosphorus atoms of oligonucleotides. To assess the viability of this process, the present work examined the Michaelis-Arbuzov-type alkylation reactions of phosphites bearing two deoxynucleosides and a suitable leaving group with aliphatic carboxylic acid-derived redox-active esters via a visible-light-driven RPC mechanism (Fig. 1C ). This reaction is believed to proceed via the nucleophilic attack of the phosphorus atom of the phosphite on the carbocation equivalent, followed by a β -elimination associated with the loss of the phosphonium species [28] . Recently, several alkylphosphonates have been prepared by electrochemical or photochemical approaches involving reactions with radicals or carbocation species and phosphites [17] , [29] , [30] , [31] . However, the phosphites that can be applied to such protocols are often limited to simple substrates such as triethyl phosphite and so the application of this concept to the chemical modification of phosphorus atoms in complex oligonucleotides has not yet been demonstrated. Development of the reaction After an extensive evaluation of reaction conditions based on our previous work [21] , [24] , the use of stoichiometric amounts of N-phenylbenzophenothiazine ( PTH1 ) and LiBF 4 was found to promote decarboxylative tertiary alkylation using a phosphite ( 1a-1 ) bearing two thymidine moieties and a 2-cyano-1-phenylethyl group as a leaving group together with a 2-phenylisobutyric acid-derived redox active ester ( 2a ). 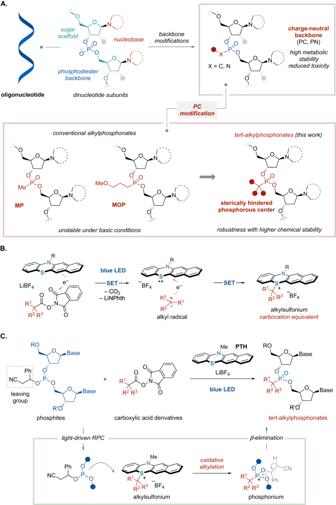Fig. 1: Chemical modification of oligonucleotides. AApplications of P–C backbones in oligonucleotide pharmaceuticals. MP methylphosphonate. MOP Methoxypropylphosphonate.BCarbocation generation via a light-driven radical-polar crossover mechanism. SET, single electron transfer.CSynthesis of oligonucleotides bearingtertiaryalkylphosphonate backbones (this work). This reaction was promoted by exposure to a blue light-emitting diode (LED) for 18 h and was performed in a mixture of acetonitrile (MeCN) and dichloromethane (DCM) to provide tertiary alkylphosphonate 3aa in a 71% yield (Table 1 , entry 1). Since phosphite 1a-1 was used as a mixture of diastereomers and each P-stereoisomer of the substrate was converted to the corresponding P-stereoisomer of the product, 3aa was obtained as a mixture of diastereomers. After separation using a silica gel column chromatography, the structure of one of the diastereomers was determined by X-ray analysis. This analysis showed that the phosphorus center had an R P conformation. Interestingly, the use of a catalytic amount of PTH1 decreased the yield (entry 2), possibly due to the low nucleophilicity of the phosphite. Table 1 Screening of leaving groups a Full size table The use of a 2-cyano-1,1-dimethylethyl leaving group ( 1a-2 ) [32] gave similar results to those of the earlier trials (Table 1 , entry 3). In contrast, a 2-cyano-1-methylethyl ( 1a-3 ) and a 2-cyanoethyl moiety ( 1a-4 ) afforded 4aa instead of the desired product 3aa (entries 4 and 5). This result indicated that deprotonation of the phosphonium intermediate generated from 1a with the simultaneous formation of a carbocation occurred at the 2ʹ-position of the ribose molecule rather than at the α-cyano position on the leaving group [33] . For this reason, a phenyl ( 1a-1 ) or 1,1-dimethyl ( 1a-2 ) substituent was expected to preferentially induce deprotonation at the α-cyano position. 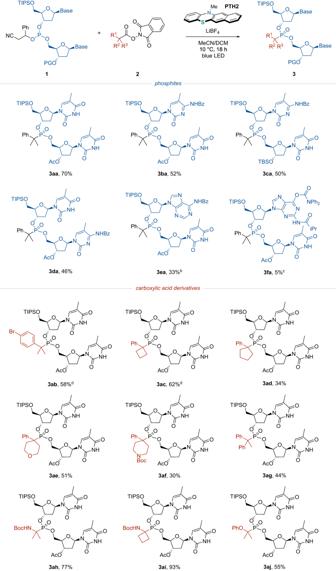Fig. 2: Substrate scope. Each reaction was carried out with1(0.05 mmol),2(0.15 mmol),PTH2(0.05 mmol) and LiBF4(0.05 mmol) in MeCN (0.3 mL) and DCM (0.2 mL) at 10 °C under blue LED irradiation for 18 ha.PTH2(1.5 equiv.), LiBF4(1.5 equiv.) and RAE (5.0 equiv.) were usedbPTH2(1.5 equiv.), LiBF4(2.0 equiv.) and RAE (5.0 equiv.) were usedc. Each reaction was carried out at 20 °C. The effects of reaction components were subsequently evaluated, using 1a-1 as the phosphite substrate (Table 2 ). Initially, various substituents were appended to the nitrogen atom on the benzo[ b ]phenothiazine. The use of N-methyl benzo[ b ]phenothiazine ( PTH2 ) slightly increased the yield while N–H benzo[ b ]phenothiazine ( PTH3 ) significantly decreased the yield (Table 2 , entries 1–3). In contrast to PTH1 , which was synthesized via a Buchwald-Hartwig amination, PTH2 could be prepared without requiring a transition metal-catalyzed amination and so this reagent is also advantageous in that respect [34] . The benzo[ b ]phenothiazine core was found to be essential to this reaction (entry 4). Table 2 Screening of reaction conditions a Full size table The effects of various additives and solvents were investigated while employing PTH2 as the redox mediator. In the absence of LiBF 4 or when this reagent was replaced by LiPF 6 or NaBF 4 , the target product was not obtained (Table 2 , entries 5–7). These results demonstrate that the presence of both Li cations and BF 4 anions was important in this reaction. The reaction proceeded in either MeCN or DCM as the sole solvent although lower yields were obtained (entries 8 and 9). The use of a more polar solvent such as DMF did not yield the desired product at all while the minimally polar solvent THF resulted in lower yields (entries 10 and 11). When the reaction temperature was lowered or raised from 10 °C, the yield was also diminished (entries 12–14). Substrate scope With the optimal reaction conditions in hand, the ranges of phosphites and redox-active esters that could be employed were investigated (Fig. 2 ). Various phosphites were initially examined together with a 2-phenylisobutyric acid derivative ( 2a ). Phosphites bearing two different 2ʹ-deoxynucleoside scaffolds such as deoxycytidine ( 3ba – 3da ), deoxyadenosine ( 3ea ) and deoxyguanosine ( 3fa ) were found to participate in this P-alkylation protocol to afford the corresponding alkylphosphonates. The relatively low yields obtained with 3ea and 3fa could possibly have resulted from the low oxidation potentials of the purine bases [35] . The reaction proceeded smoothly even with a tertiary butyldimethylsilyl (TBS) group as the 3’-OH protecting group ( 3ca ). Fig. 2: Substrate scope. Each reaction was carried out with 1 (0.05 mmol), 2 (0.15 mmol), PTH2 (0.05 mmol) and LiBF 4 (0.05 mmol) in MeCN (0.3 mL) and DCM (0.2 mL) at 10 °C under blue LED irradiation for 18 h a . PTH2 (1.5 equiv. ), LiBF 4 (1.5 equiv.) and RAE (5.0 equiv.) were used b PTH2 (1.5 equiv. ), LiBF 4 (2.0 equiv.) and RAE (5.0 equiv.) were used c . Each reaction was carried out at 20 °C. Full size image The scope of alkyl substituents was subsequently examined using 1a-1 as the nucleophile. It was found to be possible to apply aliphatic carboxylic acid derivatives with halogen substituents to the benzene ring as sites for further molecular transformations ( 3ab ) [36] . Redox-active esters with various cyclic carbon skeletons were also employed and gave the desired alkylphosphonates in good yields ( 3ac and 3ad ). In addition, heterocyclic structures such as tetrahydropyran and piperidine could be attached to the phosphorus atom ( 3ad and 3af ) and a relatively bulky diphenylmethyl group was also tolerated ( 3ag ). Furthermore, the reaction was determined to proceed without issue both at the benzylic position and at the α-positions of heteroatoms such as nitrogen and oxygen atoms ( 3ah – 3aj ). Control experiments Additional insights into this light-driven RPC protocol were obtained via a series of experiments. A stoichiometric reaction between PTH2 and 2a in the presence of LiBF 4 was initially conducted to observe the key alkylsulfonium intermediate (Fig. 3A ). Following irradiation with a blue LED for 4 h, the formation of an alkylsulfonium species was confirmed by analysis of the reaction solution using electro spray ionization–high resolution mass spectrometry. 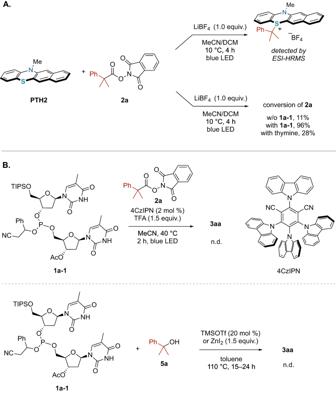Fig. 3: Control experiments. AStoichiometric reaction betweenPTH2and2a.BComparison with other protocols involving carbocation generation. 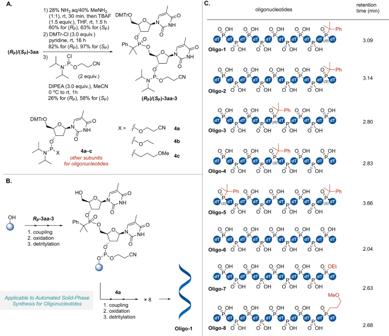Fig. 4: Application of the present method to the synthesis of oligonucleotides. ADerivatization of (RP)/(SP)-3aato give the phosphoramidites (RP)/(SP)-3aa-3.BSolid-supported automated synthesis of oligonucleotides. The synthesis ofOligo-1was exemplified.CRetention times obtained from liquid chromatography analysis of synthesized oligonucleotides. However, attempts at additional characterization by nuclear magnetic resonance spectroscopy or isolation of the alkylsulfonium were unsuccessful. Nevertheless, in the case that the reaction was performed for the same duration as used in the earlier P-alkylation reactions and with stoichiometric quantities of reagents, the majority of the original 2a was recovered. This observation prompted an investigation of the effect of the various reaction components on the conversion of 2a . In the absence of the phosphite nucleophile 1a-1 , the conversion of the redox-active ester 2a was found to be only 11% after 4 h. Conversely, after 1a-1 was added, the majority of the 2a was converted after 4 h with a 96% yield. This result suggests that 1a-1 affected the conversion of the redox-active esters. Previous reports have stated that Brønsted acids can facilitate single electron transfer from a photoredox catalyst to a redox active ester, resulting in the efficient formation of an alkyl radical [23] , [27] , [37] . Considering that the N–H group of the thymine moiety might act as a Brønsted acid, the reaction was carried out in the presence of thymine. As expected, the conversion of 2a with an increased 28% yield was observed. Fig. 3: Control experiments. A Stoichiometric reaction between PTH2 and 2a . B Comparison with other protocols involving carbocation generation. Full size image The synthetic utility of this protocol was further assessed by examining whether previously reported protocols for carbocation generation could be applied to the tertiary alkylation of 1a-1 (Fig. 3B ). The 4CzIPN-based photoredox catalysis using aliphatic redox-active esters as reported by Aggarwal and co-workers was initially employed in conjunction with 1a-1 . However, the addition of trifluoroacetic acid was found to decompose the 1a-1 such that none of the target product 3aa was obtained. Other standard methods utilizing a Lewis acid catalyst and an alcohol as the source of the alkyl group were also investigated. These trials employed trimethylsilyl trifluoromethanesulfonate or zinc iodide (ZnI 2 ) together with 2-phenyl-2-propanol ( 5a ) and 1a-1 while also heating the reaction solution [38] , [39] . Unfortunately, none of the intended product (the alkyl phosphonate 3aa ) was produced but rather a complex mixture of various compounds was generated. These results indicate that generation of the carbocation in the present protocol does not requires the addition of strong acids as mediators, which can lead to decomposition of the phosphite, thus permitting chemoselective alkylation. Automated solid-phase synthesis of oligonucleotides The synthesis of oligonucleotides having backbone structures comprising advantageous bulky alkylphosphonate dimers was also demonstrated (Fig. 4 ). Initial attempts involved the synthesis of 5ʹ-O-4,4′-dimethoxytrityl (DMTr)-phosphoramidite ( 3aa−3 ) from 3aa (Fig. 4A ), during which the isolated diastereomers ( R P )− 3aa and ( S P )- 3aa were converted to the corresponding phosphoramidites. The 5ʹ-O-acetyl and 3ʹ-O-TIPS protecting groups of 3aa were removed in series without purification to give the corresponding diols ( R P )- 3aa-1 and ( S P )- 3aa-1 . These diols were then reacted with DMTr-Cl to protect the 5ʹ-OH group and obtain the free 3ʹ-OH products ( R P )− 3aa-2 and ( S P )− 3aa-2 . Following this, a reaction with 2-cyanoethyl N,N -diisopropylchlorophosphoramidite gave phosphoramidites with R P or S P phosphorous centers for oligonucleotide synthesis [( R P )- 3aa-3 and ( S P )- 3aa-3 ]. The bulky alkylphosphonate backbone was found to remain stable in the presence of nucleophiles such as ammonia, methylamine and tetrabutylammonium fluoride (TBAF) and to be unaffected by the basic pH values imparted to the reaction solution by these amines. Fig. 4: Application of the present method to the synthesis of oligonucleotides. A Derivatization of ( R P )/( S P )- 3aa to give the phosphoramidites ( R P )/( S P )- 3aa-3 . B Solid-supported automated synthesis of oligonucleotides. The synthesis of Oligo-1 was exemplified. C Retention times obtained from liquid chromatography analysis of synthesized oligonucleotides. Full size image The solid-phase synthesis of oligonucleotides having bulky alkylphosphonate backbones was achieved by employing the widely-used phosphoroamidite method together with an automated oligo-synthesizer (Fig. 4B ) [40] , [41] , [42] , [43] , [44] . In this process, reactive phosphorus (III) compounds were incorporated into the growing oligonucleotide chain through a cycle of coupling, oxidation, and deprotection of the DMTr group steps. The synthesis cycle was repeated until the desired chain length was reached and the target oligonucleotide was then obtained through cleavage and deprotection. Using the phosphoroamidite 3aa-3 and a 5-Oʹ-DMTr-thymidine (dT)-derived phosphoroamidite bearing a 2-cyanoethoxy group ( 4a ), several oligonucleotides ( Oligo-1–6 ) were synthesized using the automated oligo-synthesizer with a solid support (Fig. 4C ). For comparison with other neutral backbones, ethyl triester-modified Oligo-7 and MOP-modified Oligo-8 were prepared from 4b and 4c , respectively. Using the optimized conditions for the synthesizer, the oligonucleotides ( Oligo-1–5 ) having bulky alkylphosphonate backbones were synthesized in the comparable yields with Oligo-6 comprising of only naturally-occurring phosphodiester backbones (Supplementary Fig. 4 ). Analysis by liquid chromatography prior to purification provided similar results in each case, confirming that there was no degradation as a consequence of the backbone structure during the solid phase synthesis or the cleavage and deprotection processes. These results confirm that the backbone structure produced in the present work was robust and that the tertiary alkylphosphonate structure was evidently unreactive in the presence of various electrophiles and acidic conditions during the solid phase synthesis. As demonstrated by the synthesis of the phosphoroamidite dimers, the oligomers also exhibited resistance to the basic conditions applied during the cleavage and deprotection processes. In addition, the product could be readily purified using a standard cartridge-type kit. Analyses by reverse phase liquid chromatography indicated that the retention time for the R P form was longer than that for the S P form, suggesting that the former was more globally hydrophobic. The retention times of Oligo-1 and Oligo-2 were also greater than those for Oligo-7 and 8 and the difference between the retention times of the S P and R P configurations of these compounds was expanded (Supplementary Fig. 4 ). The effect of chirality on global hydrophilicity/hydrophobicity was therefore increased as the molecules became larger. This effect could also modify the protein binding profiles of these compounds and lead to eutomer/distomer differences in the case that they are utilized as pharmaceuticals. The introduction of the alkyl group at the 3′ end of the oligomer had a greater effect on retention time than introduction at the center ( Oligo-1–4 ). The physicochemical and biological effects resulting from the formation of these unique tertiary alkylphosphonate backbones are currently under investigation by our group. In summary, this work demonstrated a synthetic protocol enabling the tertiary alkylation of phosphites bearing two 2ʹ-deoxynucleosides, using N-methyl benzo[ b ]phenothiazine and tertiary aliphatic carboxylic acid-derived redox-active esters in conjunction with irradiation by a blue LED. This process was found to allow the formation of bulky tertiary alkylphosphonate structures that are difficult to synthesize by conventional methods. The reaction evidently proceeds via a light-driven RPC mechanism involving carbocation species and phosphites. The resulting tertiary alkylphosphonate structures exhibit significant stability in response to various environments such that this process can be used for oligomer synthesis. The reaction in Table 2 , entry 2 is representative In a glovebox, to an oven-dried vial with a stirring bar was added PTH2 (13.2 mg, 0.05 mmol), phosphite 1a-1 (42.9 mg, 0.05 mmol), 2-phenylisobutyric acid-derived redox active ester 2a (46.4 mg, 0.15 mmol) and LiBF 4 (4.7 mg, 0.05 mmol). Then, MeCN (300 µL) and DCM (200 µL) were added to the reaction mixture. After sealing the vial with parafilm, the reaction mixture was stirred and irradiated with a 34 W blue LED with UC reactor to keep the temperature at 10 °C (Supplementary Fig. 2 ). After 18 h, the solvents were removed under reduced pressure. The crude material was then purified by flash column chromatography on silica gel (80:20:0–50:45:5, hexane/EtOAc/MeOH) to give the alkylated product 3aa (29.6 mg, 0.035 mmol, 70% isolated yield) as a white amorphous solid.